Ground-state proton transfer in the photoswitching reactions of the fluorescent protein Dronpa The reversible photoswitching between the ‘on’ and ‘off’ states of the fluorescent protein Dronpa involves photoisomerization as well as protein side-chain rearrangements, but the process of interconversion remains poorly characterized. Here we use time-resolved infrared measurements to monitor the sequence of these structural changes, but also of proton transfer events, which are crucial to the development of spectroscopic contrast. Light-induced deprotonation of the chromophore phenolic oxygen in the off state is a thermal ground-state process, which follows ultrafast (9 ps) trans – cis photoisomerization, and so does not involve excited-state proton transfer. Steady-state infrared difference measurements exclude protonation of the imidazolinone nitrogen in both the on and off states. Pump–probe infrared measurements of the on state reveal a weakening of the hydrogen bonding between Arg66 and the chromophore C=O, which could be central to initiating structural rearrangement of Arg66 and His193 coinciding with the low quantum yield cis – trans photoisomerization The “Dronpa” protein from the coral Pectiniidae [1] is a member of the class of reversibly photoconvertable fluorescent proteins, which also include mutants of Aequorea victoria green fluorescent protein (GFP) and many natural and modified GFP homologues that undergo photoisomerization reactions. In many cases, the switching reactions, which are often associated with both changes in the absorbed wavelengths as well as the fluorescence quantum yield, are both thermally and photochemically reversible [2] . The significant changes in the fluorescence quantum yield and absorption spectrum upon photoswitching allows their use in protein tracking applications in fluorescence microscopy. Dronpa undergoes photoswitching in the crystalline state, which resulted in the structural determination of the two species. Stiel et al. [3] and Wilmann et al. [4] determined the X-ray structures of the highly fluorescent on state of Dronpa, whereas Andresen et al. [5] determined the off structure. Mizuno et al. [6] performed NMR experiments of the photoswitching of Dronpa in solution, establishing photoinduced changes of the β-barrel structure. The off-state structure was cryogenically trapped after full conversion of crystals with green illumination [5] . The chromophore of Dronpa is derived from the Cys–Tyr–Gly tripeptide and is present in a cis conformation in the on state [3] , [4] , as in the A. victoria GFP [7] , [8] . Substantial structural rearrangements of the protein environment were shown to coincide with the cis – trans photoisomerization of the chromophore. In particular, Arg66 and His193 undergo large structural rearrangements, as seen in the snapshot structures of the two end products ( Fig. 1 ). These rearrangements may be linked to the low photochemical quantum yield of the on to off photoswitching reaction (3.2 × 10 −4 ( [1] , [9] )), requiring protein motion to allow relaxation in the cis – trans photoisomerization. Spectroscopic contrast is primarily developed via protonation/deprotonation of the phenolic oxygen such as that in GFP. This has been proposed to develop via excited-state proton transfer (ESPT) [9] , [10] , [11] ( Supplementary Note 1 ). 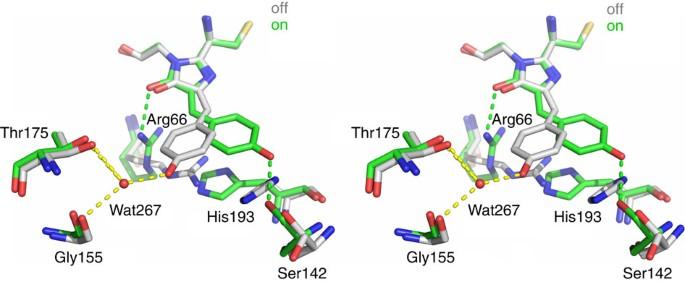Figure 1: Stereo image for overlaid coordinates for the chromophore and selected mino acids for the on (green) and off (grey) states. Structures were overlaid using all atoms for the A chain of pdb 2IOV for the on state3and 2POX for the off state5. Proposed hydrogen bonds to the chromophore are indicated to Ser142 and Arg66 in the on state3, and Gly155 and Thr175 via Wat267 for the off state5. Figure 1: Stereo image for overlaid coordinates for the chromophore and selected mino acids for the on (green) and off (grey) states. Structures were overlaid using all atoms for the A chain of pdb 2IOV for the on state [3] and 2POX for the off state [5] . Proposed hydrogen bonds to the chromophore are indicated to Ser142 and Arg66 in the on state [3] , and Gly155 and Thr175 via Wat267 for the off state [5] . Full size image A central question concerns the proposal that photoswitching of the trans off state to the bright cis on state of Dronpa involves ESPT [9] , [10] , [11] (see Supplementary Note 1 ). Photoswitching of Dronpa has been observed at the single molecule level [9] , as well as in ensembles with picosecond time resolution [10] . Transient absorption measurements in 1 H 2 O revealed a 4-ps component that was assigned to interconversion from the trans -neutral off (‘A2’) excited state to the anionic I excited state [10] . Here we probe this transition using ultrafast infrared spectroscopy and find the primary photoproduct to be the cis -neutral state instead. Although the wavelength of visible absorption, 380 nm, establishes the protonation of the phenolic oxygen in the trans off state, and a deprotonated group in the cis on form [12] , the protonation of the imidazolinone nitrogen has not been assigned for either the on or the off state. Therefore, the off state may either be neutral or cationic, and the on state may be either anionic or zwitterionic. Here we address these assignments directly from vibrational spectroscopy measurements, using the frequency of the imidazolinone C=O mode as a reporter group. The possibility of a zwitterionic chromophore has been proposed for the bright on state of a related protein asFP595. Schäfer et al. [13] , [14] propose that the ESPT in asFP595 deactivates the otherwise fluorescent zwitterionic trans chromophore, explaining the low-fluorescence quantum yield. We report the first vibrational spectroscopy measurements of Dronpa. Ultrafast infrared measurements of the off state show that the excited-state decay is linked to formation of the cis -neutral chromophore, indicating that ground-state proton transfer is slow and follows the initial photoisomerization. This is taken as evidence against ESPT in Dronpa and is in line with the absence of a significant photoacid character. We address the protonation state of the chromophore and the protein environment in the on and off states of Dronpa from Fourier-transform infrared (FTIR) difference spectroscopy. The spectra establish the cis -anionic and trans -neutral chromophore for the on and off states, respectively. Whereas no protonation differences of Glu or Asp could be demonstrated, signals belonging to Arg 66 are seen that report on the structural rearrangement that occurs concurrent with photoswitching. Ultrafast infrared measurements of the on state indicate that weakened hydrogen bonding of Arg66 to the chromophore may initiate structural rearrangements in the low quantum yield on to off switching mechanism. Equilibrium chromophore structure in the on and off states Steady-state FTIR difference measurements (see Methods section) of the on and off states identify the chromophore structures and protonation, as well as signals belonging to Arg66. The frequencies of the chromophore C=O stretching mode at 1,665/1,655 cm −1 and 1,690/1,688 cm −1 ( 1 H/ 2 H) for the on and off states, respectively, results in the definitive assignment to the cis -anionic and trans -neutral chromophore, respectively ( Fig. 2 and Table 1 ). This unambiguous assignment relies on the best characterized mode assignment, which is the localized C=O stretching mode of HBDI (4-hydroxybenzylidene-1,2 dimethylimidazolinone) and GFP spectra [15] . 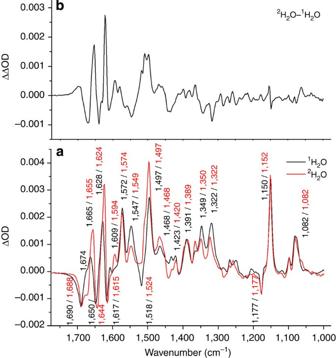Figure 2: FTIR difference spectra for the on minus off photoswitching reaction of Dronpa in1H2O and2H2O. (a) On minus off FTIR difference spectra recorded with green and blue illumination (Methods), respectively. Spectra are presented from 1,750 to 1,000 cm−1in1H2O (black) and2H2O (red). The frequencies of the major band positions are labelled in black and red accordingly. (b) Scaled double-difference spectrum for the2H2O and1H2O difference spectra. Experimental conditions were pH/pD 7.8 and 293 K. OD, optical density. Figure 2: FTIR difference spectra for the on minus off photoswitching reaction of Dronpa in 1 H 2 O and 2 H 2 O. ( a ) On minus off FTIR difference spectra recorded with green and blue illumination (Methods), respectively. Spectra are presented from 1,750 to 1,000 cm −1 in 1 H 2 O (black) and 2 H 2 O (red). The frequencies of the major band positions are labelled in black and red accordingly. ( b ) Scaled double-difference spectrum for the 2 H 2 O and 1 H 2 O difference spectra. Experimental conditions were pH/pD 7.8 and 293 K. OD, optical density. Full size image Table 1 Proposed mode assignments and frequencies of band positions in 1 H 2 O and 2 H 2 O for the on minus off FTIR difference spectra of Dronpa. Full size table Protonation of the imidazolinone nitrogen in either state (thus, considering the cis zwitterion and the trans cation for the on and off states, respectively) would result in significant upshifted frequencies of the localized C=O stretching mode, and can both be rejected. This conclusion was also verified from harmonic frequency calculations (see Supplementary Table S1 ). At p 1 H 7.8, the off state is characterized by negative bands (local minima) at 1,690, 1,650, 1,617, 1,518 and 1,177 cm −1 in 1 H 2 O, whereas the on state is characterized by phenolate chromophore bands (local maxima) with characteristic redshifted frequencies at 1,674, 1,655, 1,628, 1,609, 1,572, 1,547 and 1,150 cm −1 in 1 H 2 O ( Fig. 2 and Supplementary Fig. S1 ). The redshifted frequencies and increased intensities of the on state are characteristic for the phenolate anion, as was also previously found for the GFP [16] , [17] (see Supplementary Fig. S1 ). A comparison of the on minus off difference spectrum of Dronpa with the GFP R minus GFP A difference spectrum of GFP at 293 K [16] , [17] shows considerable similarities for both the product- and the reactant-mode frequencies and intensities (see Supplementary Fig. S1 ). The comparison allows some general conclusions, particularly with regard to the on state of Dronpa, which can be directly compared with the ‘GFP R ’ photoproduct of GFP [16] , [17] , [18] , [19] . Although the C=O stretching mode is seen at comparable frequency, the C=C and C=N modes are observed at upshifted frequency, whereas the phenol-1 mode is downshifted (see Supplementary Fig. S1 ). As discussed (see Supplementary Notes ), these band positions of the on state may be explained from the distorted non-planar configuration of the cis -anion chromophore. Assignments of the modes belonging to the off state are similarly developed from the comparison with GFP spectra, considering the difference between band positions for the neutral cis and trans chromophores, respectively ( Fig. 2 , Table 1 and see Supplementary Fig. S1 ). Bands belonging to the off as well as the on state show a distinct 1 H/ 2 H isotope substitution sensitivity ( Fig. 2 ), including the 1,547/1,549 cm −1 ( 1 H/ 2 H) bleach feature assigned to the C=N/C=C stretching mode. Similar to the on state, the possibility of protonation of the imidazolinone nitrogen, in addition to the phenolic oxygen, should be considered for the off state. However, the calculated band positions for the C=O mode of the trans anion and trans cation (see Supplementary Table S1 ) are too low and too high, respectively, to explain the experimental measurements. The band positions calculated for the trans -neutral state (see Supplementary Table S1 ) are in reasonable agreement with the proposed assignments ( Table 1 ). The 1 H/ 2 H isotope substitution effect is, however, not reproduced by harmonic frequency calculation for all modes, in particular the C=O mode, suggesting it to be more delocalized, or is modified by hydrogen bonding with the environment, potentially Arg91. There can only exist a limited number of the 3N-6 chromophore normal modes in the mid-infrared region, and additional peaks are observed ( Fig. 2 , see Supplementary Fig. S1 and Supplementary Note 2 ). Two isotope-sensitive induced absorption bands belonging to the on state may be identified as not originating from chromophore modes, at 1,674 and 1,609 cm −1 , and at 1,655 and 1,594 cm −1 in 1 H 2 O and 2 H 2 O, respectively ( Fig. 2 and Table 1 ). An assignment of the 1,674/1,655 and of the 1,609/1,594 cm −1 ( 1 H 2 O/ 2 H 2 O) bands to arginine ν asym (CN 3 H 5 + ) and ν sym (CN 3 H 5 + ) are well supported, already individually on the basis of the spectral characteristics [20] (see Supplementary Notes ). The 15 cm −1 downshift for the arginine ν sym (CN 3 H 5 + ) mode is very clearly observed owing to the isolated nature of the induced absorption band ( Fig. 2 ). Furthermore, the crystal structures of the on state (2IOV [3] ) and the off state (2POX [5] ) can be considered. As is shown in Fig. 1 , two amino acid side chains undergo dramatic structural change as a result of photoswitching, identified as Arg66 and His193. In the on state, Arg66 is hydrogen bonded to the imidazolinone carbonyl, whereas this interaction is absent in the off state. In addition, the hydrogen-bonding interaction of Arg66 with the imidazolinone carbonyl can be put forward to explain the 1 H/ 2 H substitution sensitivity of the 1,665 cm −1 C=O frequency ( Fig. 2 ). Inspection of the on state [3] and off state [5] structures suggest the Arg66 CN 3 H 5 + group to be very likely protonated in both states, in agreement with the experimental frequencies. Although the spectroscopic features already support assignment of the 1,674/1,655 and of the 1,609/1,594 cm −1 ( 1 H 2 O/ 2 H 2 O) bands to arginine ν asym (CN 3 H 5 + ) and ν sym (CN 3 H 5 + ), information from the crystal structures support the assignment to Arg66, which undergoes dramatic light-induced rearrangement. Photoswitching mechanism of the off state Time-resolved infrared measurements reveal the primary photoproduct of the off state to have a neutral trans -chromophore configuration, showing that subsequent proton transfer to finally form the on ground state is a slow, thermal ground-state process, rather than an ultrafast ESPT. Ultrafast visible (VIS)-pump infrared-probe spectroscopy of the off state of Dronpa was performed with 400 nm femtosecond excitation under conditions of photostationary accumulation with 473 nm light, allowing direct observation of the switching pathway. Pump–probe measurements directly resolve the spectral features of the primary photoproduct, which occurs with a quantum yield of ~0.3 [1] . In agreement with this estimate for the quantum yield of photoswitching, amplitude is resolved on the order of 30% for the ground-state bleach (GSB) features in the 1,580–1,715 cm −1 spectral window for a long-lived photoproduct state ( Fig. 3 ). 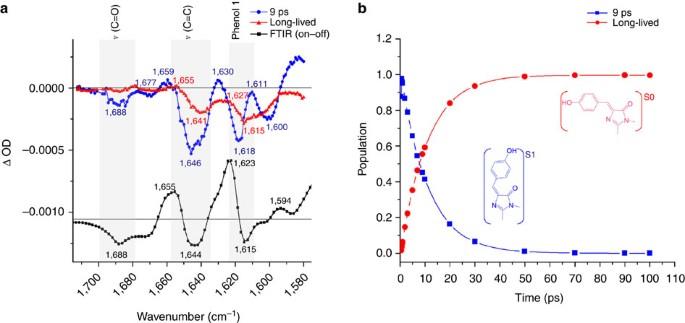Figure 3: Ultrafast VIS-pump infrared-probe spectroscopy of the off state of Dronpa at 6,100 nm, accumulated under continuous illumination at 473 nm. (a) Pump-on minus pump-off transient absorption data were collected in a single spectral window from 1,575 to 1,715 cm−1, with delays up to 100 ps. To accumulate the off state, the sample was continuously illuminated with 25 mW continuous-wave illumination at 473 nm, and was physically moved to replace the sample on a shot-to-shot basis. Presented are the difference spectra for a sequential model showing the spectra associated with the two dominant time constants present, at 9 ps and a long-lived photoproduct at 100 ps. For comparison, the corresponding portion of the static FTIR difference spectrum in2H2O, offset by 0.007 OD, is shown in the same region, plotted as the ‘on minus off’ difference spectrum to match the direction of the negative bands belonging to the off state. (b) Time traces of the relative amplitudes of the spectra shown in panela, including global fit with a single 9 ps time constant. OD, optical density. Figure 3: Ultrafast VIS-pump infrared-probe spectroscopy of the off state of Dronpa at 6,100 nm, accumulated under continuous illumination at 473 nm. ( a ) Pump-on minus pump-off transient absorption data were collected in a single spectral window from 1,575 to 1,715 cm −1 , with delays up to 100 ps. To accumulate the off state, the sample was continuously illuminated with 25 mW continuous-wave illumination at 473 nm, and was physically moved to replace the sample on a shot-to-shot basis. Presented are the difference spectra for a sequential model showing the spectra associated with the two dominant time constants present, at 9 ps and a long-lived photoproduct at 100 ps. For comparison, the corresponding portion of the static FTIR difference spectrum in 2 H 2 O, offset by 0.007 OD, is shown in the same region, plotted as the ‘on minus off’ difference spectrum to match the direction of the negative bands belonging to the off state. ( b ) Time traces of the relative amplitudes of the spectra shown in panel a , including global fit with a single 9 ps time constant. OD, optical density. Full size image A single time constant is sufficient to globally fit the transient absorption data from 1,715 to 1,580 cm −1 up to 100 ps, providing two sequential states. A 9-ps time constant is followed by a long-lived product state that has constant amplitude up to 100 ps ( Fig. 3 ). The 9-ps component has bleach features at 1,688, 1,646, 1,618 and 1,600 cm −1 , with induced absorption at 1,659, 1,630 and 1,583 cm −1 . For comparison, the on minus off FTIR difference spectrum is included, shown to coincide bleach features belonging to the off state. The 1,688 (−)/1,677 (+) cm −1 feature may be assigned to the chromophore C=O mode, where the reduced bond order is taken as the basis for the assignment of the downshifted induced absorption in the singlet excited state. The GSB band positions are the same for the C=O, the C=C and the phenol-1 modes in the 9-ps spectrum and the FTIR difference spectrum at 1,688, 1,644–1,646 and 1,618 cm −1 , respectively. Notably, the 1,600 (−)/1,583 (+) cm −1 difference band is not seen in the FTIR difference spectra and is tentatively assigned on the basis of its intensity to the phenol 2 mode ( Table 1 and Fig. 2 ). The 9-ps component is assigned to the decay of the singlet excited state of the neutral trans chromophore, in agreement with previous fluorescence measurements [9] . Habuchi et al. [9] reported a 14-ps time constant for fluorescence measurements of the off state of Dronpa in 1 H 2 O at pH 7.4, with excitation at 390 nm and detection at 440 nm. After the excited-state decay a photoproduct is formed, which has a reduced amplitude for the GSB, in addition to showing downshift of the maxima to 1,641 and 1,615 cm −1 , indicative of the formation of upshifted but weak induced absorptions for the C=C and phenol-1 modes ( Fig. 3 , Supplementary Fig. S2 and Supplementary Note 3 ). The photoproduct is stable for the 100-ps observation time of the pump–probe data, much longer than the reported 14 ps fluorescence lifetime, definitively supporting assignment to a ground-state intermediate that is structurally distinct from both the on and off states [9] . The comparison of the long-lived component with the static FTIR difference spectra exclude the possibility of deprotonation. Explicitly, spectral signatures for the anionic cis chromophore, in particular the upshifted C=C and phenol-1 frequencies seen at 1,655 and 1,623 cm −1 in the static FTIR difference spectra ( Fig. 2 and Supplementary Fig. S1 ), are strikingly absent from the long-lived photoproduct spectrum ( Fig. 3 ). It is therefore shown that deprotonation of the phenolic oxygen occurs on time scales much longer than 100 ps as a thermal ground-state process, which also involves reformation of the Arg66 and His193 interactions and conformations, and results in eventual formation of the anionic cis chromophore in the on state ( Fig. 1 ). This demonstrates the central conclusion that proton transfer occurs thermally on the ground-state surface on the way to the on ground state. As the electronic configuration is assigned to a singlet ground state, the chromophore has isomerized to the cis configuration at the exocyclic double bond. Transient infrared measurements are thus inconsistent with ESPT, which was proposed on the basis of a small 1 H/ 2 H kinetic isotope effect that was determined from transient visible absorption spectroscopy [10] . Another proposal made on the basis of quantum chemistry calculations put forward the ESPT, but in a concerted fashion together with trans – cis photoisomerization [12] , [21] , which is also not supported by our measurements. Li et al. [12] , [21] argued that ESPT and the trans – cis photoisomerization would either act as competing channels or occur simultaneously in the off to on switching, whereas our observations show a sequential process in which the ground-state deprotonation follows the initial ultrafast trans – cis photoisomerization reaction ( Fig. 3 ). The origin of the apparent 1 H/ 2 H kinetic isotope effect on the ultrafast component remains to be resolved [10] . However, Habuchi et al. [9] reported a 14-ps decay constant for fluorescence measurements of the off state of Dronpa in 1 H 2 O, in contrast to Fron et al. [10] who reported a 4-ps time constant in 1 H 2 O from transient absorption. Blue excitation of the off state does not result in absorption differences of the arginine ν asym (CN 3 H 5 + ) and ν sym (CN 3 H 5 + ) bands up to 100 ps ( Fig. 3 ) as seen in the on state ( Fig. 4 ). This agrees with the absence of the hydrogen-bonding interaction of the Arg66 (CN 3 H 5 + ) group to the chromophore C=O in the off state [5] , and suggests that the side-chain reorganization to reform the on state proceeds on a time scale longer than 100 ps ( Fig. 5 ). 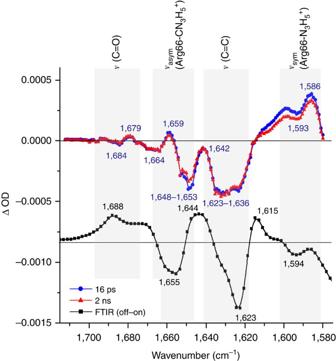Figure 4: Ultrafast VIS-pump infrared-probe spectroscopy of the on state of Dronpa at 6,100 nm. Pump-on minus pump-off transient absorption data was collected in a single spectral window from 1,575 to 1,715 cm−1, with delays up to 1 ns. Presented are the difference spectra for a sequential model, showing the spectra associated with the two dominant time constants present, at 16 and 2 ns. For comparison, the corresponding portion of the static FTIR difference spectrum in2H2O, offset by 0.007 OD, is shown in the same region, plotted as the off minus on difference spectrum to match the direction of the negative bands belonging to the on state. OD, optical density. Figure 4: Ultrafast VIS-pump infrared-probe spectroscopy of the on state of Dronpa at 6,100 nm. Pump-on minus pump-off transient absorption data was collected in a single spectral window from 1,575 to 1,715 cm −1 , with delays up to 1 ns. Presented are the difference spectra for a sequential model, showing the spectra associated with the two dominant time constants present, at 16 and 2 ns. For comparison, the corresponding portion of the static FTIR difference spectrum in 2 H 2 O, offset by 0.007 OD, is shown in the same region, plotted as the off minus on difference spectrum to match the direction of the negative bands belonging to the on state. OD, optical density. 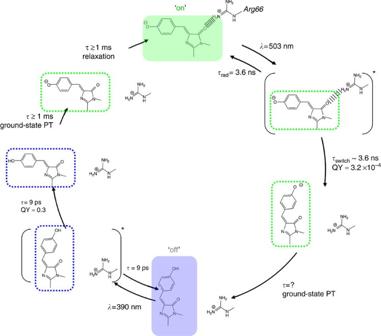Figure 5: Proposed assignments and photoswitching reaction path for the on and off states of Dronpa. Electronic excited states are indicated with an asterisk (*) character and put between brackets. The weakened hydrogen bonding between the Arg66 (CN3H5+) group and the chromophore imidazolinone C=O group is indicated with an increased distance in the excited state on the on conformation. Conditions are p1H/2H 7.8 and 293 K. Full size image Figure 5: Proposed assignments and photoswitching reaction path for the on and off states of Dronpa. Electronic excited states are indicated with an asterisk (*) character and put between brackets. The weakened hydrogen bonding between the Arg66 (CN 3 H 5 + ) group and the chromophore imidazolinone C=O group is indicated with an increased distance in the excited state on the on conformation. Conditions are p 1 H/ 2 H 7.8 and 293 K. Full size image In the off state, the crystal structure has modelled a water molecule A267 at 2.50 Å distance from the phenolic oxygen, thought to be in a protonated state. Water A267 is in turn hydrogen bonded to the carboxylate of Glu144 at a distance of 3.06 Å [22] . This may suggest that a situation exists in Dronpa, which is similar to GFP [23] , which stabilizes the protonated form of the phenolic oxygen via electrostatic repulsion from the carboxylate group. It has also been proposed as a possible route for ESPT [9] . However, our FTIR measurements exclude the possibility of stable protonation changes of glutamate or aspartate from the absence of induced absorption in the ~1,710/1,720 cm −1 ( 1 H/ 2 H) region ( Fig. 2 ). Similarly, the transient infrared absorption changes, measured in 2 H 2 O, do not reveal signal in the 1,710 cm −1 spectral region ( Fig. 3 ), arguing against the possibility of transient protonation of Glu 144 in the 9-ps component. Photoswitching mechanism of the on state As the photoswitching quantum yield of the on state is 3.2 × 10 −4 ( [1] , [9] ), pump–probe measurements do not directly observe the switching pathway but reveal the vibrational response of the radiative state. Indirect information on the photoswitching pathway is, however, obtained from establishing the excited-state structural response. Ultrafast VIS-pump infrared-probe spectroscopy of the on state of Dronpa was performed in the 1,570–1,715 cm −1 spectral region, with 503 nm femtosecond excitation, and delays up to 1 ns ( Fig. 4 ). The measurements were globally fitted, requiring two time constants, 16 ps and 2 ns. Both the time constants were associated with approximately equal amplitude, and no significant spectral differences were present ( Fig. 4 , Supplementary Fig. S3 and Supplementary Note 4 ). With data extending only up to 1 ns, the 2-ns time constant is not well determined, but is considered to belong to the fluorescence lifetime, taken to be 3.6 ns [9] . The spectra are assigned to the biphasic decay of the singlet excited state of the cis -anionic chromophore, which is the dominant decay reaction in the on state. The data are compared with the off minus on FTIR difference spectra, which coincides the position of the major GSB peak for the ‘C=C’ mode at 1,624 cm −1 in the FTIR difference spectrum, with the pump-on minus pump-off difference spectra belonging to both the 16 ps and 2 ns phases ( Fig. 4 ). As the FTIR difference spectrum shows a side band at the high-frequency side, the GSB band shape of the 16 ps and 2 ns components is considered to arise from a heterogeneous ground-state population, which underlies the main bleach region from 1,623 to 1,636 cm −1 . Consistent with a reduced cross section and downshifted frequency relative to the trans -neutral chromophore, the 1,664 (−)/1,659 (+) cm −1 feature may contain the contributions from the imidazolinone C=O mode. This would fit the interpretation that the 1,655 cm −1 band belonging to the on state in 2 H 2 O has contributions from both the chromophore C=O as well as the ν asym (CN 3 H 5 + ) from Arg66 ( Table 1 ). The 1,593 (−)/1,586 (+) cm −1 band in both the 16-ps and 2-ns components may be assigned to the ν sym (CN 3 H 5 + ) of Arg66, as the bleach feature coincides with its band position in the on state ( Fig. 2 and Table 1 ). The frequency downshift observed for the singlet excited state of the on state of Dronpa signals a weakening of the hydrogen-bonding interaction with the chromophore imidazolinone C=O group. This key observation may be at the basis of the on to off switching of Dronpa, which involves rearrangement of the side chain of Arg66. Similarly, contribution of the ν asym (CN 3 H 5 + ) mode would be expected in the 1,664–1,648 cm −1 region ( Fig. 4 ). Following this interpretation, an upshifted feature 1,648 (−)/1,659 (+) cm −1 may conversely report on the reduced hydrogen bonding to the chromophore C=O group. Harmonic frequency calculations of the Arg side chain in the presence and absence of a hydrogen-bonded water molecule indicate the ν asym (CN 3 H 5 + ) frequency to upshift by 7 cm −1 (from 1,696 to 1,702 cm −1 at the density functional theory (DFT) B3LYP/6-311+g(d,p) level), whereas the ν sym (CN 3 H 5 + ) downshifts by 6 cm −1 (from 1,694 to 1,688 cm −1 ; not shown). The small 1,684 (−)/1,679 (+) cm −1 feature might arise from other protein C=O groups. The weakened hydrogen bonding to the chromophore imidazolinone C=O group in the excited state may report on charge relocation or, alternatively, ultrafast geometrical rearrangement of the chromophore. In particular, it is noted that CASSCF calculations indicated that in contrast to the planar cis chromophore [24] , [25] , twisted geometries invert the direction of charge migration from the imidazolinone to the phenol ring [25] , which may correspond to the observed ~7° angle between the phenolate and imidazolinone rings in the ground-state crystal structure of the on state [3] . From the vibrational spectroscopy analysis, the on state is definitively assigned as the anion. Photoisomerization is known to occur with a low quantum yield, given as 3.2 × 10 −4 ( [9] ). The crystal structure analysis has shown that amino acid side chains of Arg66 and His193 adopt entirely different conformations after photoswitching, in addition to breaking and creating hydrogen bonding to the phenolic oxygen after photoisomerization (Fig. 1 ) [3] , [5] . Andresen et al. [5] proposed a sequence of rearrangements following the cis – trans photoisomerization of the chromophore. It was argued that both Arg66 and Val157 sterically hinder the phenolic ring in the trans configuration, but Andresen et al. [5] proposed Val157 movement as a first step. However, the Arg66 side chain in the off state effectively replaces the His193 position in the on state, and thus relocation of His193 must come before or simultaneously with relocation of Arg66 side chain ( Fig. 1 ). Moreover, the new His193 position in the off state sterically clashes with the phenolic ring in the on state, making this argument circularly permutated. Therefore, a more likely model is the simultaneous, or concerted, motion of Arg66 and His193 together with excited-state cis – trans isomerization of the chromophore. The low quantum yield of 3.2 × 10 −4 ( [9] ), together with the 3.6 ns excited-state lifetime suggests an estimate for the intrinsic time constant of 11 μs for the thermal ground-state structural rearrangements. The observation of weakening of the hydrogen bonding of Arg66 with the chromophore C=O group, which persists for the duration of the radiative state, is suggested to be the first step towards the (low probability) concerted switching mechanism. Therefore, we put forward a three-state model for photoswitching from the on to the off state ( Fig. 5 ), from the measurements of the radiative state ( Fig. 4 ). The first intermediate is the singlet excited state that weakens the hydrogen bonding to Arg66, followed by concerted cis – trans isomerization and rearrangement of Arg66 and His193. Photoisomerization is proposed to be followed by thermal ground-state proton transfer to the phenolic oxygen to form the neutral trans chromophore in the off state ( Fig. 5 ) In summary, we present infrared spectroscopy measurements on the response of the chromophore and surrounding protein environment in the photoswitching reactions of Dronpa. These establish the chromophore deprotonation and protonation in the off and on photoswitching reactions to occur as thermal ground-state processes. Importantly, we definitively assign the primary photoproduct of the off state to be a ground-state neutral cis chromophore, thus excluding the possibility of ESPT. The thermal deprotonation of phenolic oxygen develops significant spectroscopic contrast, which is crucial for practical applications such as super-resolution imaging. For the on state, observation of reduced hydrogen bonding between the chromophore and Arg66 in the photoswitching precursor state presages the rearrangements that are linked to photoswitching. FTIR spectroscopy The expression plasmid pRSETb-Dronpa was kindly provided by A. Miyawaki (Riken Brain Science Institute, Tokyo, Japan). Dronpa was expressed and purified as previously described [3] . The purified protein was concentrated to 1.3 mM in 1 H 2 O Tris buffer (5 mM Tris, 20 mM NaCl, pH 7.8) and 2 H 2 O samples were prepared by repeated concentration and dilution in a 2 H 2 O Tris buffer (5 mM Tris, 20 mM NaCl, pD 7.8). Evaluation of the isotope substitution of the solvent from the absolute FTIR spectra of the samples showed better than 95% replacement. The concentrated protein sample was inserted between calcium fluoride windows in a Harrick cell (Harrick Scientific Products) with a 12-μm Teflon spacer to give an optical density of 1.2 Abs at 503 nm and absolute infrared absorption of 0.9 in the amide I region. Steady-state FTIR difference measurements were recorded on a Bio-Rad FTS 175C FT-IR spectrophotometer equipped with an mercury cadmium telluride (MCT) detector, and collected at 4 cm −1 resolution. The sample was repeatedly photoconverted between the on and off states by illumination with a bright white-light source (KL2500LCD), with 495 nm high-pass filter (ThorLabs FGL495; 500 mW total power in a 2-inch diameter spot) and 405–410 nm high-power light-emitting diode (700 mA, 3.9 V, 5 W, Mouser Electronics 897-LZ110UA00-U8; 100 mW total power in a 2-inch diameter spot). The illumination periods for green and blue light were 20 and 10 min, respectively; this is an extensive period to ensure full conversion to the off and on states. The repeatability of the infrared spectral differences were on the order of 2% of the dominating amplitude differences, and 1,800 and 1,200 scans were averaged for 1 H 2 O and 2 H 2 O, respectively. The signal-to-noise ratio, particularly in the 1,600–1,700 cm −1 region, was optimized by adjusting the dissolved protein concentration and path length to yield an absolute absorption value of 0.8–0.9 at 1,650 cm −1 , having contributions from both amide I and 1 H 2 O absorption. The final difference spectra were generated by averaging of multiple individual measurements. Optical power measurements were done with ThorLabs S310C. Ultrafast VIS-pump/mid-infrared-probe spectroscopy The output of Ti:Sapphire regenerative amplifier (Spitfire PRO, Spectra Physics, 4 W, 70 fs) was divided between two optical parametric amplifiers (Topas, Light Conversion). One of the parametric amplifiers was equipped with non-collinear difference, frequency-generation module that enabled wavelength tuning in mid-infrared region. The other used additional frequency mixing stages to generate ultraviolet and visible light pulses. The mid-infrared-probe beam was attenuated by neutral density filter and split in two to produce signal and reference beams. Signal beam was focused onto the sample with off-axis parabolic mirror into a spot of 75 μm diameter full-width at half maximum. Transmitted signal and reference beams were directed to spectrometers (Triax190, Horiba) with the MCT array detectors (Infrared associates) and the FPAS data acquisition systems (Infrared Systems Development Corp.). The two MCT arrays consisted of 128 pixels each 0.2 mm in width and 0.5 mm in height, and with a 50-μm spacing between active areas. The uniformity among the pixels was specified better than 15% with typical D *-values of 30–40 × 10 9 cm Hz 1/2 W −1 (peak value at 9 μm, 1 kHz). All measurements described in this paper were performed at 6.1 μm centre-probe wavelength and a spectrometer resolution of 1.2 cm −1 . Water vapour and polystyrene thin-film absorption was used to fine tune the calibration of the acquired spectra. Consequently, the spectral calibration of the FTIR measurements (described above) and dispersive femtosecond spectroscopy measurements were matched to better than 1 cm −1 . The ultraviolet and VIS-pump beam was modulated with an optical chopper at 500 Hz (at half of pulse repetition rate of the laser), and its timing relative to probe pulse was changed with delay line. The pump-beam intensity was adjusted using reflective neutral density filters, and the polarization was rotated to a ‘magic angle’ (54.7°) relative to the probe beam. Finally, it was focused on the sample to 300 μm spot full-width at half maximum. This corresponded to an average power density of 1.8 W cm −2 in the 503-nm pump case and to 4.2 W cm −2 in the 400-nm pump case. A custom-built sample translator was used to move the sample cell in Lissajous patterns at an average speed of 50 μm ms −1 . By adjusting the translation speed, it was possible to change the number of pump pulses hitting the same sample spot. Pump-on minus pump-off difference spectra were obtained by shot-to-shot referencing and on the fly-signal discrimination to reject outliers. Transient absorption measurements were analysed by global analysis, using a previously reported ultrafast spectroscopy modelling toolbox [26] . Data treatment included the fitting of instrument response function (about 100 fs) and chirp, and applied a sequential model, using coupled differential equations, to retrieve the species-associated difference spectra relative to the ground state, which correspond to the dominant time constants that describe the full time-resolved data set. How to cite this article: Warren, M. M. et al. Ground-state proton transfer in the photoswitching reactions of the fluorescent protein Dronpa. Nat. Commun. 4:1461 doi: 10.1038/ncomms2460 (2013).